Vanadium disulfide flakes with nanolayered titanium disulfide coating as cathode materials in lithium-ion batteries Unlike the vast majority of transition metal dichalcogenides which are semiconductors, vanadium disulfide is metallic and conductive. This makes it particularly promising as an electrode material in lithium-ion batteries. However, vanadium disulfide exhibits poor stability due to large Peierls distortion during cycling. Here we report that vanadium disulfide flakes can be rendered stable in the electrochemical environment of a lithium-ion battery by conformally coating them with a ~2.5 nm thick titanium disulfide layer. Density functional theory calculations indicate that the titanium disulfide coating is far less susceptible to Peierls distortion during the lithiation-delithiation process, enabling it to stabilize the underlying vanadium disulfide material. The titanium disulfide coated vanadium disulfide cathode exhibits an operating voltage of ~2 V, high specific capacity (~180 mAh g −1 @200 mA g −1 current density) and rate capability (~70 mAh g −1 @1000 mA g −1 ), while achieving capacity retention close to 100% after 400 charge−discharge steps. Transition metal dichalcogenides (TMDs) are an emerging class of two-dimensional (2D) materials with chemical formula of MX 2 , where M denotes a transition metal (e.g., Mo, W, Re, etc.) and X represents a chalcogen (e.g., S or Se) [1] , [2] . Recently there has been intense research activity directed towards deploying TMD materials for electrochemical energy storage applications [3] , [4] , [5] . However most of the commonly used TMDs such as molybdenum disulfide (MoS 2 ) and tungsten disulfide (WS 2 ) are semiconductors with low electrical conductivity, which limits their usefulness as battery materials. Deployment of such TMDs as electrodes is only possible when they are mixed with highly conductive carbon-based materials. However, this greatly reduces the active material loading and limits the high-rate capability of the electrode. In contrast, vanadium disulfide (VS 2 ) is a conducting TMD material [6] and exhibits metallic behavior (Supplementary Fig. 1 ). Therefore, VS 2 -based electrodes could in principle be deployed in lithium (Li)-ion batteries without requiring a high content of conductive carbon additives or conductive binders, which are inactive materials. In spite of this promise, the realization of VS 2 -based electrodes [7] , [8] , [9] , [10] , [11] in Li-ion batteries has been limited by its poor stability, which leads to low cycle life. In the literature, volume expansion leading to pulverization [7] is cited as a reason for poor stability of VS 2 in Li-ion batteries. To buffer the volume expansion, VS 2 is mixed with mechanically resilient carbon materials (e.g. graphene) to create a composite electrode that offers improved stability [7] . Here, we demonstrate that VS 2 flakes can be stabilized in the electrochemical environment of a Li-ion battery by simply coating them with a few nm thick layer of titanium disulfide (TiS 2 ). In our approach, densely packed VS 2 flakes with high crystallinity are grown directly on the surface of a carbon nanotube current collector substrate by chemical vapor deposition (CVD). Then a conformal TiS 2 coating is deposited on the VS 2 platelets by atomic layer deposition (ALD). Electrochemical testing as well as in situ optical as well as ex situ scanning electron microscopy (SEM) observation reveal a pronounced stability enhancement for the TiS 2 -coated VS 2 as compared to bare VS 2 . First-principles density functional theory (DFT) calculations indicate that unlike VS 2 which undergoes large Peierls distortion during lithiation/delithiation, the TiS 2 lattice remains relatively undisturbed. Consequently, the TiS 2 coating provides an electrochemically and mechanically stable support that “buttresses” the VS 2 platelets and prevents the underlying VS 2 sheets from delaminating and peeling off the surface. To our knowledge, the role of Peierls distortion (during lithiation/delithiation) in promoting the failure of VS 2 electrodes has not been identified in the past, and thus constitutes a key contribution of this work. The resultant VS 2 -TiS 2 structures are remarkably resilient and offer a striking enhancement in stability over the baseline VS 2 electrode in Li-ion batteries. In fact, the performance of the TiS 2 protective coating is superior to ALD deposited layers of metal oxides (e.g. Al 2 O 3 , ZrO 2 , TiO 2 ) [12] , fluorides (e.g. AlF 3 ) [13] , and nitrides (e.g. TiN) [14] that have been used to passivate different electrode surfaces. Deposition of such condensed and electrically insulating films induces low Li-ion diffusivity and electron transport, and thus suppresses initial capacity and rate capability [15] . In fact, such capacity quelling effects have been reported even for extremely thin (few angstroms thick) ALD deposited coatings. The TiS 2 coating on the other hand does not suppress the specific capacity or the rate capability of VS 2 . This we presume is because TiS 2 is also a TMD material and is compatible with VS 2 . Moreover, TiS 2 is conductive and shares a similar electronic structure (Supplementary Fig. 1 ) as VS 2 , which allows the high-rate capability performance of VS 2 to be retained despite being sandwiched by TiS 2 layers. Synthesis and characterization A densely packed forest of VS 2 sheets was grown (Methods) on a carbon nanotube current collector substrate (Supplementary Fig. 2 ) by a dual-zone atmospheric pressure chemical vapor deposition (APCVD) process (schematically represented in Fig. 1a ). Since metal halide precursors [16] tend to offer better growth regulation and reproducibility when compared to metal oxides, we have selected the chloride reactant (VCl 3 ) and S powder as precursors for CVD growth. In addition, ~5% H 2 was incorporated into the carrier gas in the CVD reactor in order to generate more active species (e.g., VCl − , VCl 2 − ) from the vanadium precursor molecules. This enhances the nucleation site density and growth rate of the VS 2 flakes. A carbon nanotube (CNT) film was selected as the current collector substrate because of its light weight, high conductivity and flexibility. The VS 2 platelets are observed predominantly on the surface of the CNT film. An examination of the junction (Supplementary Fig. 3 ) between the VS 2 and CNT substrate indicates that the VS 2 platelets are embedded (or lodged) into the CNT current collector. This is important since it indicates a strong interface and good electrical connectivity between the VS 2 flakes and the CNT current collector substrate. Fig. 1 Synthesis and characterization of VS 2 and VS 2 -TiS 2 flakes. a Schematic of the procedure for fabricating VS 2 and VS 2 -TiS 2 composites. b , c Top-view SEM ( b : scale bar = 10 μm; c : scale bar = 3 μm) of VS 2 flakes with different magnification. d , e Top-view SEM ( d : scale bar = 10 μm; e : scale bar = 1 μm) of the VS 2 -TiS 2 structures with different magnification. f Raman spectrum of VS 2 and VS 2 -TiS 2 . g X-ray diffraction pattern of VS 2 and VS 2 -TiS 2 flakes Full size image After the VS 2 growth was completed, ALD was used to deposit a nanolayered TiS 2 coating over the VS 2 platelets (VS 2 -TiS 2 ) by using TiCl 4 and S as precursors (Methods). The morphologies of the as-synthesized VS 2 and VS 2 -TiS 2 structures are revealed by top-view SEM imaging as shown in Fig. 1b−e . In Fig. 1b , densely packed micrometer scale VS 2 flakes can be seen growing vertically off the current collector. The smooth flakes of regular hexagon or semi-hexagon shape (Fig. 1c ) suggest their high crystallinity. The ALD-deposited TiS 2 faithfully replicates the nanoforest structure and flake shape of the VS 2 due to the excellent conformability and precise thickness control of the ALD technique (Fig. 1d ). Note that there is a roughening (Fig. 1e ) of the VS 2 flakes post TiS 2 deposition which is attributed to the polycrystalline phase of ALD TiS 2 . The elemental distribution results obtained by EDS elemental mapping (Supplementary Figs. 4 – 5 ) further confirm the homogeneous distribution of V, S and V, S, Ti atoms on the surfaces of VS 2 and the VS 2 -TiS 2 structures, respectively. X-ray photoelectron spectroscopy (XPS) also provided confirmation of the VS 2 and TiS 2 phase (Supplementary Fig. 6 ). To evaluate the electrical conductivity of the VS 2 and VS 2 -TiS 2 flakes, electrical transport measurements were performed on individual flakes (Supplementary Fig. 7 ). Due to the two-dimensional morphology of the flakes, the sheet resistance [17] was used to compare the conductivity of the VS 2 and VS 2 -TiS 2 flakes. The sheet resistance ( R s ) of the VS 2 flake is in the 200–900 Ω ⎕ −1 range, while that of the VS 2 -TiS 2 flake lies in the 500–2400 Ω ⎕ −1 range. After TiS 2 deposition, the conductivity of the VS 2 flake has decreased, but is still comparable to pure VS 2 . These results indicate that the intrinsic high electrical conductivity of VS 2 is retained in the VS 2 -TiS 2 architecture. The VS 2 and VS 2 -TiS 2 flakes were further characterized by Raman spectroscopy (Fig. 1f ). We observe Raman peaks of VS 2 at 263, 304, and 379 cm −1 . The peaks at 263 and 379 cm −1 correspond to the E 1g and A 1g modes of VS 2 and are comparable to previous reports [16] , [18] for CVD grown VS 2 . In our experiments, we also observed an additional peak at 304 cm −1 , which we attribute to an in-plane sliding mode ( E ′) for VS 2 that can arise due to interlayer mismatch [19] . ALD coating of TiS 2 on VS 2 introduced a new peak at 324 cm −1 which corresponds [20] , [21] , [22] to the A 1g mode of TiS 2 . Other peaks exhibit similar position and width indicating that the VS 2 structure was well preserved after the ALD process. X-ray diffraction (XRD) analysis also confirmed the crystallinity of the as-grown VS 2 and VS 2 -TiS 2 flakes (Fig. 1g ). It should be noted that in the literature [7] , [16] , [18] , [23] , [24] , [25] , [26] , [27] there is large scatter in the Raman data for VS 2 . 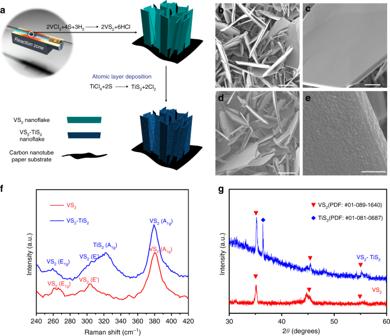Fig. 1 Synthesis and characterization of VS2and VS2-TiS2flakes.aSchematic of the procedure for fabricating VS2and VS2-TiS2composites.b,cTop-view SEM (b: scale bar = 10 μm;c: scale bar = 3 μm) of VS2flakes with different magnification.d,eTop-view SEM (d: scale bar = 10 μm;e: scale bar = 1 μm) of the VS2-TiS2structures with different magnification.fRaman spectrum of VS2and VS2-TiS2.gX-ray diffraction pattern of VS2and VS2-TiS2flakes This is illustrated in Supplementary Table 1 . These differences arise due to the growth method (i.e., CVD vs. hydrothermal synthesis), laser (polarization) set-up, flake curvature as well as poor environmental stability when VS 2 Raman measurements are taken under atmospheric conditions (Supplementary Fig. 8 ). These effects are discussed in detail in the Supplementary Information . Raman spectra of the CNT substrate before and after the depositions are provided in Supplementary Fig. 9 . The G band at ~1580 cm −1 is attributed to vibration of sp 2 bonded carbon atoms in the CNT, while the D-band (~1350 cm −1 ) is attributed to defects and disorder in the CNT [28] . The ratio of the intensity of the D to G band ( I D / I G ) of the pristine CNT film is ~0.45. This value is increased to ~0.6 after deposition. This slight increase in CNT defectiveness is presumably due to the high temperature and aggressive chemical environment related to the use of halogen precursors. There is also a higher frequency shoulder to the G band (D′ band ~1620 cm −1 ); this shoulder becomes more prominent after deposition. Also, a new peak at ~1438 cm −1 appeared post deposition, which is related to other carbonaceous materials [29] . Transmission electron microscopy (TEM) was performed to probe the structure of the synthesized VS 2 and VS 2 -TiS 2 flakes. The flake edges appear to be roughened (Fig. 2a, c ) after the TiS 2 ALD deposition, which is consistent with the SEM observations in Fig. 1e . High-resolution TEM (HRTEM) imaging of VS 2 is shown in Fig. 2b . The inset of Fig. 2b shows the corresponding fast Fourier transform (FFT) pattern. The well-defined spots in the FFT pattern indicates the single-crystal structure of the VS 2 sheet planes viewed along the [010] zone axis. Some visible spots in the FFT are labeled as (102), \(\left( {\bar 10\bar 2} \right)\) , (002), \(\left( {00\bar 2} \right)\) , (100), and \(\left( {\bar 100} \right)\) . The measured reciprocal spacing G (100) measured = 2.24 Å −1 using the calibration scale bar matches well with the calculated theoretical G (100) theoretical = 2.25 Å −1 . The real space spacing d 100 = \((\sqrt 3 /2)\) a = 2π/ G (100), where a is the lattice constant. The extracted value of a ≈ 3.24 Å is consistent with the bulk lattice constant (3.221 Å) of VS 2 (PDF: #01-089-1640). It is noted that weaker spots about 10° next to the (102) and \(\left( {\bar 10\bar 2} \right)\) spots were observed in the FFT pattern. This is likely due to the rotation of the stacked multilayer VS 2 structure during growth. 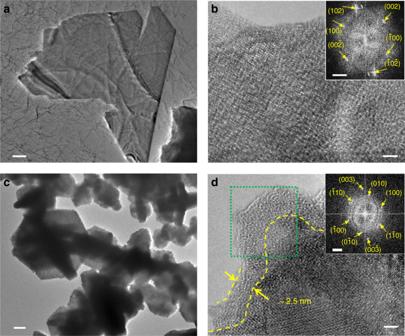Fig. 2 TEM and HRTEM characterization of VS2and VS2-TiS2.aTEM (scale bar = 200 nm) andbHRTEM image (scale bar = 2 nm, inset shows the corresponding FFT pattern (scale bar = 2 nm−1)) of a typical VS2flake.cTEM (scale bar = 200 nm) anddHRTEM image (scale bar = 2 nm, inset shows the FFT pattern (scale bar = 2 nm−1) of the region within the green box) of a typical VS2-TiS2flake. TEM transmission electron microscopy, HRTEM high-resolution transmission electron microscopy, FFT Fast Fourier Transform Figure 2d shows HRTEM imaging of a VS 2 -TiS 2 flake. ALD of TiS 2 introduced a ~2.5-nm-thick layer on the surface. The inset in Fig. 2d is the FFT pattern from a selected region indicated by the green dashed box in the HRTEM image. Many spots from VS 2 still can be identified, for example, (100), (010), \((1\bar 10)\) and (003), but there are more spots in ring-like contrast that is consistent with polycrystalline TiS 2 . FFT of other VS 2 -TiS 2 flakes were analyzed and similar results were obtained. These confirm the existence of the TiS 2 polycrystalline phase. Fig. 2 TEM and HRTEM characterization of VS 2 and VS 2 -TiS 2 . a TEM (scale bar = 200 nm) and b HRTEM image (scale bar = 2 nm, inset shows the corresponding FFT pattern (scale bar = 2 nm −1 )) of a typical VS 2 flake. c TEM (scale bar = 200 nm) and d HRTEM image (scale bar = 2 nm, inset shows the FFT pattern (scale bar = 2 nm −1 ) of the region within the green box) of a typical VS 2 -TiS 2 flake. TEM transmission electron microscopy, HRTEM high-resolution transmission electron microscopy, FFT Fast Fourier Transform Full size image Electrochemical properties To evaluate the electrochemical performance of the VS 2 and VS 2 -TiS 2 electrodes, coin cells were assembled (Methods). The galvanostatic charge–discharge voltage profiles of the VS 2 and VS 2 -TiS 2 electrodes between 1.5 and 3.5 V (vs. Li/Li + ) at a current density of ~200 mA g −1 are shown in Fig. 3a . The electrochemical intercalation and removal of Li in VS 2 can be described by the following reaction: \(x{\mathrm{Li}}^ + + xe^ - + {\mathrm{VS}}_2 \leftrightarrow {\mathrm{Li}}_x{\mathrm{VS}}_2\) . The voltage plateau in the discharge/charge curve at about 2 V is indicative of the transition from the α-VS 2 to the β-Li x VS 2 phase [7] . The lithiated Li x VS 2 phase shows promise as a cathode material in Li-ion batteries. It is noteworthy that the TiS 2 surface coating does not suppress the specific capacity of VS 2 . As Fig. 3a indicates both the bare VS 2 and the VS 2 -TiS 2 core-shell electrode delivers a similar initial (i.e. first cycle) specific capacity of about 180 mA h g −1 . For the VS 2 electrode, the mean operating voltage is at ~2.3 V. After TiS 2 coating, the operating voltage of the VS 2 -TiS 2 electrode dropped to ~2.1 V. One reason for this might be the lattice stress caused by TiS 2 growth on the surface of the VS 2 flake, which may affect the intercalation and de-intercalation potential of lithium ions into VS 2 . Moreover, it has been commonly observed that ALD-coated layers affect lithium diffusion and electron transport processes [12] , [30] , which could also influence the charge−discharge voltage profiles. Fig. 3 Electrochemical characterization. a The galvanostatic charge–discharge voltage profiles of the VS 2 electrode and VS 2 -TiS 2 electrode between 1.5 and 3.5 V (vs. Li/Li + ) at a current density of 200 mA g −1 . b Rate performance of the VS 2 and VS 2 -TiS 2 electrodes. c Cycling performance and Coulombic efficiency of VS 2 electrode and VS 2 -TiS 2 electrode at 200 mA g −1 . d Capacity retention of VS 2 electrode and VS 2 -TiS 2 electrode at 1000 mA g −1 . e Comparison of the VS 2 -TiS 2 electrode (starred) with other commonly used cathodes [ 7 , 37 , 38 , 39 , 40 , 41 , 42 , 43 , 44 , 45 , 46 , 47 , 48 , 49 ] in Li-ion batteries. The y -axis on the plot gives the specific capacity achieved by the cathode material at the completion of a specified number of charge−discharge cycles given on the x -axis of the plot. The charge−discharge rate (or current density) at which the electrode is cycled is also specified next to each data point on the plot Full size image The rate performances of the VS 2 and VS 2 -TiS 2 electrodes was investigated as shown in Fig. 3b . Since TiS 2 is metallic (Supplementary Fig. 1 ) similar to VS 2 , the conductivity of VS 2 -TiS 2 is still comparable to that of pure VS 2 (Supplementary Fig. 7 ). Consequently, the overall rate performance of the VS 2 electrode was not significantly affected by the TiS 2 coating. The results show that the baseline VS 2 and the VS 2 -TiS 2 electrode exhibits a capacity above 150 and 180 mA h g −1 , respectively in the first five cycles at a current density of ~200 mA g −1 . Even when the current density is increased to ~2000 mA g −1 (~10C charge−discharge rate), a specific capacity of ~40 mA h g −1 is achieved, which indicates that the VS 2 -TiS 2 electrode is capable of high C-rate operation. The cyclic stability of the samples was investigated at a current density of ~200 mA g −1 , as shown in Fig. 3c . The VS 2 -TiS 2 electrode demonstrated excellent cycle stability above 180 mA h g −1 after 100 charge−discharge steps, while the baseline VS 2 electrode under the same conditions exhibits a rapid capacity loss. We also investigated the cycling performance of the electrodes at a higher current density of ~1000 mA g −1 (see Fig. 3d ). The capacity retention rate is close to ~100% for the VS 2 -TiS 2 electrode after 400 continuous cycles of charge and discharge, while the capacity retention of the baseline VS 2 electrode was only ~40% under the same test conditions. The charge and discharge voltage profiles for the VS 2 and VS 2 -TiS 2 electrodes for the 1st, 100th, 200th, 300th and 400th cycles are provided in Supplementary Fig. 10 . From the charge−discharge profiles, it is evident that the stability of the electrodes has been significantly improved by the TiS 2 coating. Moreover, the over-potential between charge and discharge did not amplify with cycling in the VS 2 -TiS 2 electrode, which is quite different from the pristine VS 2 electrode for which the over-potential continues to increase with cycling. 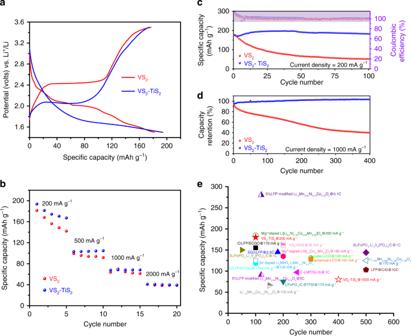Fig. 3 Electrochemical characterization.aThe galvanostatic charge–discharge voltage profiles of the VS2electrode and VS2-TiS2electrode between 1.5 and 3.5 V (vs. Li/Li+) at a current density of 200 mA g−1.bRate performance of the VS2and VS2-TiS2electrodes.cCycling performance and Coulombic efficiency of VS2electrode and VS2-TiS2electrode at 200 mA g−1.dCapacity retention of VS2electrode and VS2-TiS2electrode at 1000 mA g−1.eComparison of the VS2-TiS2electrode (starred) with other commonly used cathodes [7,37,38,39,40,41,42,43,44,45,46,47,48,49] in Li-ion batteries. They-axis on the plot gives the specific capacity achieved by the cathode material at the completion of a specified number of charge−discharge cycles given on thex-axis of the plot. The charge−discharge rate (or current density) at which the electrode is cycled is also specified next to each data point on the plot Figure 3e compares the VS 2 -TiS 2 performance with the other cathodes that are commonly used in Li-ion batteries. At low current densities (~200 mA g −1 ), the VS 2 -TiS 2 electrode provides a very high specific capacity of over 180 mA h g −1 (after 100 charge−discharge cycles) which is among the best results reported to date. Moreover, unlike many of the other cathode materials, the VS 2 -TiS 2 electrode can also be operated at high charge−discharge rates and provides a capacity of ~70 mA h g −1 (after 400 cycles) at a current density of ~ 1000 mA g −1 . In the reported literature, only lithium iron phosphate (LFP)-based cathodes provide higher specific capacities at comparable charge−discharge rates. Note that these results are reported for a realistic mass loading (~ 3.5 mg cm −2 ) of the VS 2 -TiS 2 material. In situ optical characterization In order to monitor structural changes during lithiation and delithiation, we carried out in situ observation of an individual VS 2 and VS 2 -TiS 2 flake during the charge−discharge process. The schematic of the optical transparent cell is shown in Fig. 4a with the VS 2 (or VS 2 -TiS 2 flake) as the device cathode and Li metal as the anode. The cell was sealed using a transparent glass cover (Supplementary Fig. 11 ), through which in situ observation of structural changes during lithiation and delithiation could be performed. To better monitor the structure change, we chose relatively thinner flakes of ~20 nm in thickness (Supplementary Fig. 12 ). The freshly sealed VS 2 or VS 2 -TiS 2 flake showed an open circuit voltage at around 2.6 V vs. Li/Li + . We carried out lithiation by gradually decreasing the cathode potential to 1.5 V (vs. Li/Li + ). Subsequently, the cathode potential was increased to 3.5 V (vs. Li/Li + ), to complete the delithiation process. Voltage profiles for the VS 2 and VS 2 -TiS 2 cells are shown in Supplementary Fig. 13 . Note that the gap between the electrodes is much larger for the in situ cell as compared to a coin cell, which lead to a higher over-potential (Supplementary Fig. 13 ). Fig. 4 Observations of structural changes to the VS 2 and VS 2 -TiS 2 flakes during the lithiation and delithiation process. a Schematic of transparent cell set-up for in situ optical imaging. b − d Optical images of VS 2 flake at the original status, lithiation status, and delithiation status. Scale bar = 20 μm. e − g Optical images of VS 2 -TiS 2 flake at the original status, lithiation status, and delithiation status. Scale bar = 20 μm. The color difference of the background shown in ( b − d ) and ( e − g ) was caused by using a different light source of the optical microscope. h Ex situ SEM image (scale bar = 10 μm) of VS 2 flakes after galvanostatic charge−discharge cycling at 1000 mA g −1 for 400 cycles. i Corresponding SEM image (scale bar = 3 μm) of VS 2- TiS 2 flakes after galvanostatic charge−discharge cycling at 1000 mA g −1 for 400 cycles. SEM scanning electron microscopy Full size image As shown in Fig. 4b−d , for the pure VS 2 flake, we observe significant changes in the color and morphology of the flake under the optical microscope. During the lithiation process (Fig. 4c ), partial transparency appeared on the original VS 2 flake, and this change was not reversible when carrying out the delithiation process. In fact, the transparency spreads over the entire VS 2 flake, indicating significant permanent (irreversible) change or damage to the flake. In stark contrast to this, with the TiS 2 coating, there is no obvious color or structural change to the VS 2 -TiS 2 flake as shown in Fig. 4e−g . The reflection light intensity contrast, which is the reflection from the 2D flake compared with that from the substrate, is related to the absorption of the 2D flake. The observed transparency spreading can thus be understood as a decrease in the overall absorption of the VS 2 flake. Since uncoated VS 2 is not stable during lithium intercalation, it likely undergoes delamination, which effectively decreases the overall absorption and hence induces the observed transparency. This interpretation is confirmed by the completely different behavior of TiS 2 -coated VS 2 . The TiS 2 -coated VS 2 is stable during the lithium intercalation process and we expect the thickness of the VS 2 flake remains unchanged. The reflection contrast of the TiS 2 -coated VS 2 flake, therefore, remains unchanged during and after the lithium intercalation, consistent with our observation. Ex situ SEM characterization These results were also corroborated by ex situ SEM imaging of the flakes. For this, we opened the coin cells (tested in Fig. 3d ) that were cycled for 400 charge−discharge steps inside a glove box. The VS 2 and VS 2 -TiS 2 electrodes were extracted from the coin cells, and SEM was used to observe the morphology of these electrodes. As shown in Fig. 4i , no obvious change in the morphology can be observed for the VS 2 -TiS 2 electrode. These observations are consistent with the in situ optical imaging and indicate that with the help of the TiS 2 coating, the structural integrity of the VS 2 could be maintained during electrochemical cycling. 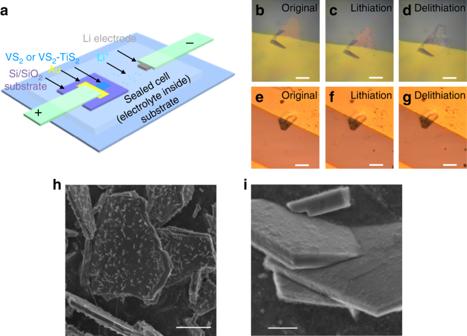Fig. 4 Observations of structural changes to the VS2and VS2-TiS2flakes during the lithiation and delithiation process.aSchematic of transparent cell set-up for in situ optical imaging.b−dOptical images of VS2flake at the original status, lithiation status, and delithiation status. Scale bar = 20 μm.e−gOptical images of VS2-TiS2flake at the original status, lithiation status, and delithiation status. Scale bar = 20 μm. The color difference of the background shown in (b−d) and (e−g) was caused by using a different light source of the optical microscope.hEx situ SEM image (scale bar = 10 μm) of VS2flakes after galvanostatic charge−discharge cycling at 1000 mA g−1for 400 cycles.iCorresponding SEM image (scale bar = 3 μm) of VS2-TiS2flakes after galvanostatic charge−discharge cycling at 1000 mA g−1for 400 cycles. SEM scanning electron microscopy In contrast, SEM imaging of the bare VS 2 electrode revealed a multitude of VS 2 flakes delaminating and peeling off (see Fig. 4h ) the surface of the electrode, confirming structural damage during cycling, which is responsible for the fast capacity fade. First principles calculations Density functional theory calculations were carried out (Methods) to obtain a fundamental understanding of lithiation/delithiation in and out of the VS 2 and VS 2 -TiS 2 structures. The calculations are not for a single sheet, rather all calculations assumed a bulk structure. That is, the out-of-plane lattice constants were chosen so that it minimized the free energy of bulk Li 2 VS 2 and bulk Li 2 TiS 2 . The dynamics of an individual Li-ion can be described as a series of migrations between adjacent transition metal sites belonging to the same MS 2 (M = V or Ti) layer. Each of these migrations requires that an adjacent Li site be vacant. It therefore follows that the migration of a Li-ion is also the migration of a vacancy in the opposite direction. To model these migrations, we remove a Li-ion from a fully intercalated system, leaving behind a single Li vacancy. We then use the climbing-image nudged elastic band method (CNEB) to calculate the energy barrier associated with moving a Li-ion from an adjacent site into that vacancy. 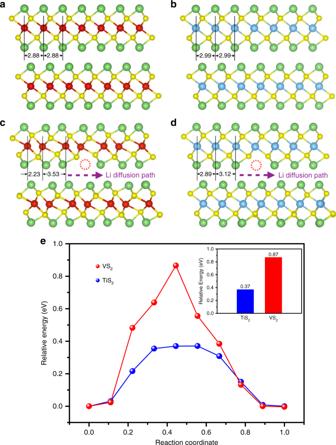Fig. 5 DFT calculations. Fully intercalated pristine layered structures,aLi2VS2andbLi2TiS2. Here, the yellow and green balls symbolize sulfur and lithium atoms, respectively. Vanadium atoms are red and titanium atoms are blue. Lithium diffusion in these systems requires that a neighboring lithium site is vacant. The corresponding intercalated structures with Li vacancies, marked with dashed red circles are shown forcLi2VS2anddLi2TiS2. Lithium diffusion paths are indicated by purple arrows. Notice that the even spacing of 2.88 Å between vanadium atoms in fully intercalated Li2VS2distort to 2.23 and 3.53 Å when a lithium vacancy is introduced. The distortion is much smaller in Li2TiS2, for which the distances between titanium atoms distort from 2.99 Å to 2.89 Å and 3.12 Å.eEnergy profile along the lithium diffusion path in the VS2and TiS2(inset indicates the energy barriers for lithium migration). Reaction coordinates 0 and 1 correspond to the beginning and end of the lithium migration paths, which are equilibrium systems, while noninteger reaction coordinates in-between denote the fraction of the lithium migration path that has been traversed. DFT density functional theory Figure 5e compares the energy profiles of these migration processes in VS 2 and TiS 2 . Clearly, VS 2 is associated with a much larger energy barrier for migration. This is because VS 2 and TiS 2 respond very differently to the presence of a Li vacancy. Specifically, VS 2 layers “Peierls distort” when a vacancy is introduced, so that the V atoms are alternatingly pinched and pulled apart (Fig. 5a, c ). When a Li migrates, the VS 2 distortion must reverse its phase, i.e., the pinched atoms separate, while the pulled atoms converge. This rearrangement has an energy cost which is reflected in VS 2 ’s tall energy profile (Fig. 5e ). Meanwhile, the fully intercalated TiS 2 crystal is much less susceptible to distortion, in that we see very little deviation from the pristine structure when a vacancy is introduced (Fig. 5b, d ). As a result, the TiS 2 crystal remains relatively undisturbed during the migration process. This can explain why the TiS 2 coating dramatically improves the lifetime of the VS 2 cathode. Through repeated charging and discharging cycles, periodic agitation to the host VS 2 material can cause degradation over time. With TiS 2 coating, the robust outermost layers endure much less disturbance during Li migration. As a result, the outer TiS 2 is resilient to the charging/discharging cycles, while the inner VS 2 layers are more protected from degradation due to the mechanical support provided by the TiS 2 coating. Fig. 5 DFT calculations. Fully intercalated pristine layered structures, a Li 2 VS 2 and b Li 2 TiS 2 . Here, the yellow and green balls symbolize sulfur and lithium atoms, respectively. Vanadium atoms are red and titanium atoms are blue. Lithium diffusion in these systems requires that a neighboring lithium site is vacant. The corresponding intercalated structures with Li vacancies, marked with dashed red circles are shown for c Li 2 VS 2 and d Li 2 TiS 2 . Lithium diffusion paths are indicated by purple arrows. Notice that the even spacing of 2.88 Å between vanadium atoms in fully intercalated Li 2 VS 2 distort to 2.23 and 3.53 Å when a lithium vacancy is introduced. The distortion is much smaller in Li 2 TiS 2 , for which the distances between titanium atoms distort from 2.99 Å to 2.89 Å and 3.12 Å. e Energy profile along the lithium diffusion path in the VS 2 and TiS 2 (inset indicates the energy barriers for lithium migration). Reaction coordinates 0 and 1 correspond to the beginning and end of the lithium migration paths, which are equilibrium systems, while noninteger reaction coordinates in-between denote the fraction of the lithium migration path that has been traversed. DFT density functional theory Full size image To extend the generality of our study, we also investigated partially intercalated systems (Supplementary Fig. 14 ), which contains one Li per unit of VS 2 or TiS 2 . We found that LiVS 2 Peierls distorts in a manner similar to what we found in Li 2 VS 2 . Meanwhile, the distortion in LiTiS 2 is imperceptible (Supplementary Fig. 14 ), as it was in Li 2 TiS 2 . Note that the cathode likely contains regions of both LiVS 2 and Li 2 VS 2 , resulting in an intermediate capacity as observed in the experiments. These results suggest that the distortion of Li-intercalated VS 2 appears at various intercalation concentrations, and therefore occurs throughout the entire charge/discharge process. By contrast, Li-intercalated TiS 2 remains resilient to distortion, suggesting that the TiS 2 coating can protect the inner VS 2 through the complete charge−discharge cycle. Since DFT indicates that TiS 2 offers superior stability compared to VS 2 , then would a bulk TiS 2 flake be superior to VS 2 -TiS 2 ? While TiS 2 is a metal, it is ~4.5 times less conductive than VS 2 . Reported electrical conductivity value for VS 2 [18] is ~3000 S cm −1 compared to ~676 S cm −1 for TiS 2 [31] . For ~2.5 nm TiS 2 coating, this is not a significant limitation (Supplementary Fig. 7 ), but for thicker TiS 2 flakes, the lower conductivity can limit performance, especially for fast charging and high power applications. For this reason, the VS 2 -TiS 2 electrode is preferred to only TiS 2 or only VS 2 . Lastly, we used DFT to investigate the binding strength of lithium with pure VS 2 and VS 2 with a coating layer of TiS 2 . Our calculations indicate that the binding energy of lithium to the second layer of fully charged, pure VS 2 is 3.12 eV. By replacing the top layer of VS 2 with TiS 2 , this binding energy is slightly reduced to 3.09 eV. Assuming that binding energies should result in more residual lithium trapped in the material after the recharging process, we can use these energies to estimate the ratio of lithium occupation in both materials after delithiation. The canonical distribution of statistical mechanics predicts this ratio to be: \({{R}} = e^{ - \Delta E/k_{\mathrm{B}}T}\) , where Δ E is the difference in formation energies, k B = 8.62 × 10 −5 eV K −1 is Boltzmann constant, and T = 293 K is the room temperature. Inserting Δ E = 3.13 − 3.09 = 0.03 eV, we estimate that the residual lithium occupation in pure VS 2 to be about three times greater than that of VS 2 with the TiS 2 coating. As a result, we expect that delithiation, and therefore the recharging of the battery, is more complete with the TiS 2 coating. This result also indicates that the presence of TiS 2 improves the capacity retention of the battery during charge−discharge cycles. To summarize, we have demonstrated a procedure to stabilize VS 2 cathodes in Li-ion batteries, based on coating with TiS 2 . Electrochemical testing, in situ optical imaging and first principles DFT calculations indicate that the stability of the battery is drastically improved after the VS 2 core is encapsulated by a thin (~2.5 nm) TiS 2 coating layer. SEM imaging of the VS 2 electrode post cycling indicates that VS 2 layers tend to delaminate (i.e., peel off) the surface of the bulk VS 2 flake. This is to be expected as structural distortion due to Li intercalation and extraction will have the greatest negative impact on the outermost VS 2 layers. These layers are the least protected and the most vulnerable. The VS 2 sheets within the bulk of the flake are mechanically supported (buttressed) by neighboring sheets and are therefore far less likely to detach or separate from the flake. Therefore supporting the outermost VS 2 layers close to the surface becomes critical, which is what the ~2.5 nm-thick TiS 2 coating is able to accomplish. Since there is minimal lattice distortion to the TiS 2 coating, the TiS 2 layer remains intact on the VS 2 flake. Its presence prevents the underlying VS 2 layers from delaminating from the surface of the flake, in spite of the large lattice distortion and volume changes that these underlying layers will encounter on lithiation and delithiation. In this way, the presence of TiS 2 at the surface preserves the structure of VS 2 and prevents the delamination and break-up of the VS 2 material during the lithiation−delithiation process. These findings provide new opportunity for the rational design of conductive TMD materials for building high-performance Li-ion batteries. VS 2 growth on the carbon current collector by CVD Dual-zone APCVD was utilized for the synthesis of vanadium disulfide (VS 2 ) sheets on the carbon nanotube current collector. As shown in schematic Fig. 1a , the source boats containing vanadium trichloride (VCl 3 ) and sulfur (S) powders were arranged within a quartz tube in the furnace tube, where VCl 3 was located at the center of the furnace, while S was placed ~25 cm upstream. The substrate which is about 14 mm × 75 mm × 0.02 mm (W × L × H) faced downward on the top edge of the source boat containing VCl 3 . Since the ratio between vanadium and sulfur was critical to achieving the suitable stoichiometry, the evaporation of VCl 3 and S powders were independently controlled by two temperature zones. In the optimized growth condition, a quartz boat containing ~0.1 g VCl 3 powders (Sigma-Aldrich) was placed in the center of the first furnace zone, and a quartz boat containing ~0.6 g S powders (Sigma-Aldrich) was positioned in the center of the second furnace zone. Both boats were semi-cylindrical cuts from a quartz tube without vertical edges along the direction of flow, which allows for more even downstream flow of the precursor materials to the substrates. Before the growth, the quartz tube was baked at ~120 °C and purged with ~80 sccm forming gas (nitrogen mixed with ~5% hydrogen) for ~1 h. Then, the heating zone 1 with the VCl 3 boat was heated to ~750 °C at a rate of ~80 °C/min. The temperature of the S boat during growth was ~250 °C. When the VCl 3 temperature reached ~750 °C, the gas flow was reduced to ~50 sccm. After ~10-min growth of VS 2 under atmospheric pressure, the flow rate was increased to ~80 sccm again and the system was naturally cooled down to room temperature over ~2.5 h. TiS 2 ultrathin layer coating by ALD The VS 2 sample was loaded in the ALD chamber for polycrystal TiS 2 coating at ~400 °C. A solid-precursor-cylinder containing S powder was connected to the ALD system for sulfur supply, while titanium tetrachloride (TiCl 4 ) was used as the titanium (Ti) precursor. To maintain the high vapor pressure of both precursors, the temperature of the solid-precursor-cylinder and TiCl 4 cylinder were maintained at ~400 °C and ~30 °C, respectively. The base pressure of the system was ~900 mTorr by using Ar as the carrier gas (~100 sccm). The ALD growth cycle consisted of ~10 s S pulsing + ~30 s Ar purging + ~5 s TiCl 4 pulsing + ~30 s Ar purging. One hundred cycles yielded ~2 nm thick polycrystal TiS 2 coating (VS 2 -TiS 2 ) with the deposition rate of ~0.02 nm/cycle. Surface and crystal structure characterizations The structure of the materials (VS 2 -TiS 2 and VS 2 ) was investigated by SEM (Carl Zeiss Supra field-emission scanning electron microscope). Energy-dispersive X-ray spectroscopy (EDS) in conjunction with SEM analysis and Raman spectroscopy measurements were conducted to obtain the surface elemental information. The Raman measurements were performed with a lab-made micro Raman spectrometer. To prevent possible oxidation of vanadium disulfide caused by laser irradiation, the samples were mounted in an optical cryostat covered by a quartz window with an internal pressure of ~7×10 −7 Torr. The 532 nm laser with a spot size of ~2 μm and intensity of ~5 mW (LRS-0532 DPSS, Laserglow Technologies, Canada) was irradiated on the sample through the quartz window. The reflected signal was obtained and analyzed by a high-speed spectroscopy CCD camera (iDus 420 Series, Andor Technology Ltd, UK) and imaging spectrometer (Shamrock 500i, Andor Technology Ltd, UK). The resolution of the Raman system is ~0.6 cm −1 . The step size used in measurements was ~1.34 cm −1 . All spectra were collected by integrating the signal for ~60 s. A Tecnai TF-30 transmission electron microscope (FEI, Hillsboro, OR) was used to study the crystal structure of synthesized flakes and the surface distribution of TiS 2 layer. Focused ion beam (FIB) imaging was performed on an FEI Helios Nanolab 600i dual beam electron microscope. The FIB was conducted with gallium ions operating at 30 kV and electron imaging was performed at 15 kV. XPS was carried out using Al Kα radiation (~1486 eV) in a PHI 5000 Versaprobe TM system with a hemispherical analyzer and an 8-channel detector. XRD was done in a PANalytical X’Pert Pro Diffractometer. Electrochemical measurements The electrochemical properties of the VS 2 flakes without/with TiS 2 coating as cathode materials in Li-ion batteries were evaluated by a galvanostatic charge/discharge technique. Coin cells (2032-type) were used to assemble test cells in an Ar-filled glove box (MBraun Labstar). The electrodes (VS 2 , VS 2 -TiS 2 ) and current collector were cut to the desired shape without binder or additional conductive additives. The mass loading of the composite was ~3.5 mg cm −2 and the capacity was normalized on the total mass of the electrodes. Metallic lithium was used as the counter/reference electrode. A total of ~30 μL of ~1 M lithium bis(trifluoromethanesulfonyl)imide in 1,3-dioxolane and 1,2-dimethoxyethane (1:1 by volume) with ~0.1 mol L −1 LiNO 3 additive was used as the electrolyte. Charge−discharge measurements were carried out galvanostatically at various current densities over a voltage range of 1.5 to 3.5 V (vs. Li/Li + ) using an Arbin BT2000 battery testing system. In situ optical observation A designed transparent cell was built for in situ optical observation during the lithiation−delithiation process. For this, the VS 2 flakes grown by APCVD were transferred onto an SiO 2 /Si substrate (~300 nm SiO 2 ) by simple tapping. VS 2 nanoflakes on the substrate with a lateral size of ~30 µm were targeted by optical microscopy. Next a shadow mask with grids of ~80 µm were applied on the top to deposit the Au pattern by e-beam evaporation, so as to partially cover the flake. The patterned sample that acts as the cathode in the Li-ion cell was then transferred into the glove box for the device assembly. A Li anode, the patterned VS 2 or VS 2 -TiS 2 cathode and the liquid electrolyte were encapsulated within a transparent enclosure. The anode and cathode materials were in contact with stainless steel meshes that served as the current collectors for the battery. A cover glass was placed on top of the central region and the electrolyte was filled into this region. The visualization cell, including cut outs for the current collectors were sealed using epoxy (Supplementary Fig. 11 ). Density functional theory simulation Calculations utilized plane-wave DFT with projector augmented-wave (PAW) pseudopotentials as implemented in the Vienna ab initio Simulation Package (VASP) [32] . The generalized gradient approximation (GGA) was employed using the Perdew−Burke−Ernzerhof functional [33] , for which van der Waals interactions were considered using density functional methods of optB86 [34] , [35] . Ionic relaxation calculations used a plane-wave basis set including energies up to 550 eV. We assume that, when fully lithiated, the bulk TMD crystals can hold two Li for each unit of MS 2 (M = Ti or V), with one Li bound above and one below each transition metal atom. Hence, we denote the intercalated TMD by the chemical formula Li 2 MS 2 . For the primitive bulk cells of Li 2 VS 2 and Li 2 TiS 2 , the Brillouin zone was sampled with a Γ-centered Monkhorst−Pack mesh of dimensions 11 × 11 × 4. Relaxation iterations persisted until all interatomic Hellmann−Feynman forces settled below 0.01 eV Å −1 for all atoms, while the self-consistent field iterations ceased when the changes in both total energy and the eigenvalues settled below 10 −6 eV between iterations. Calculations involving cathode surfaces included 16 Å of vacuum separation to eliminate interactions between periodic adjacent cells. Larger amounts of vacuum produced nearly identical ground state energies. During the discharging process, the intercalated Li evacuate the crystal, traveling in-plane between the MS 2 layers towards the crystal’s edge via successive migrations to unoccupied Li sites. The activation energies required for these migration were calculated using the nudged elastic band method combined with the climbing-image technique [36] . For these calculations, a Li vacancy is placed in an otherwise fully intercalated 4 × 4 × 2 supercell, while eight intermediate images are used to describe its migration to an adjacent site. In addition, the formation energies of dilithiation of a single layer were calculated using; E form = E int − E vac − 2 × E Li , where E int , E vac , and E Li are the free energies of a fully intercalated system, a system with one layer of Li removed, and an isolated Li + ion. The binding energies are then the additive inverses of the free energies. Lastly, to extend the generality of our study, we investigated lithiation and delithiation in partially intercalated TMDs, which contains one Li per unit of MS 2 and is denoted as LiMS 2 . We removed one Li from an otherwise pristine 4 × 4 × 2 LiMS 2 , and allowed the system to relax, respecting the same convergence criteria as described above.